A viral peptide that targets mitochondria protects against neuronal degeneration in models of Parkinson’s disease Mitochondrial dysfunction is a common feature of many neurodegenerative disorders, notably Parkinson’s disease. Consequently, agents that protect mitochondria have strong therapeutic potential. Here, we sought to divert the natural strategy used by Borna disease virus (BDV) to replicate in neurons without causing cell death. We show that the BDV X protein has strong axoprotective properties, thereby protecting neurons from degeneration both in tissue culture and in an animal model of Parkinson’s disease, even when expressed alone outside of the viral context. We also show that intranasal administration of a cell-permeable peptide derived from the X protein is neuroprotective. We establish that both the X protein and the X-derived peptide act by buffering mitochondrial damage and inducing enhanced mitochondrial filamentation. Our results open the way to novel therapies for neurodegenerative diseases by targeting mitochondrial dynamics and thus preventing the earliest steps of neurodegenerative processes in axons. The progressive loss of structure and function of neurons in neurodegenerative diseases, including Parkinson’s disease (PD), involves mitochondrial dysfunction and early axonal degeneration [1] , [2] , [3] . Accordingly, agents that could protect mitochondrial functions may have broad therapeutic implications, especially considering that we still lack efficient therapies to block neuronal demise in the early stages of neurodegeneration. Viruses, as obligatory parasites, have evolved highly specific means to hijack cellular pathways. To optimize the survival in their host, many viruses express factors that block or delay the death of infected cells, by acting notably at the mitochondrial level, thereby suppressing one of the most ancient antiviral mechanisms [4] . For neurotropic viruses, protecting infected neurons from excessive damage or death makes theoretical sense to facilitate viral spread and persistence, given the poor regenerative capacity of neurons. For instance, rabies virus neurovirulence is inversely correlated with its capacity to kill infected neurons [5] . In addition, delayed axonal degeneration in slow Wallerian degeneration ( Wld s ) mutant mice has been shown to favour infection by neurotropic viruses that spread in the central nervous system (CNS) using axonal transport [6] . This has led to the hypothesis that some virally encoded products may be used as tools to retard or suppress neurodegeneration [7] , [8] . Ideally, however, such tools should target axonal degeneration, which has been shown to precede cell body death in various neurodegenerative diseases, notably PD [3] . The identification of factors able to retard axonal degeneration may therefore come from the study of viruses that replicate while causing minimal damage to neurons. A case in point is Borna disease virus (BDV), a neurotropic RNA virus that persists in the brain of many animal species without causing damage to neurons [9] . BDV non-cytolytic replication depends on the expression of an 87 amino acids viral protein called X [10] . This non-structural protein was initially described as an important regulator of viral RNA synthesis and of polymerase complex assembly in the nucleus of infected cells [11] , [12] , [13] . Later, it was shown that X represents the first mitochondrion-localized protein of an RNA virus that inhibits rather than promotes induction of apoptosis, thereby favouring non-cytolytic viral persistence [10] and escape to mitochondrial antiviral signalling protein-mediated host cell defence [14] . It was therefore tempting to investigate whether the X protein could protect neurons against neurodegenerative insults. In this study, we examine the capacity of BDV infection, as well as of the isolated expression of the X protein, to protect against mitochondrial respiratory complex I toxins, which induce oxidative stress and neurodegeneration [15] , [16] , [17] . We use oriented primary cultures of neurons grown in microfluidic chambers to demonstrate that the X protein displays selective and strong axoprotective properties. We also report that the isolated expression of the X protein is able to protect dopaminergic neurons of the nigrostriatal pathway from degeneration in a mouse model of PD. In addition, we find that the neuroprotection conferred by the X protein results from enhanced mitochondrial filamentation. Finally, we identify a cell-permeable peptide derived from the X protein that recapitulates all our findings obtained with the full-length protein. Importantly, in vivo neuroprotection with this peptide can be achieved upon intranasal administration, thereby opening the way to novel therapies for neurodegenerative diseases. BDV protects from rotenone-induced axonal fragmentation To test the neuroprotective potential of BDV infection upon a direct axonal or somatic insult, we used oriented primary neuronal cultures grown in microfluidic devices, which permit the strict physical separation and fluidic isolation of somatodendritic and axonal compartments. Consistent with our previous findings [18] , [19] , [20] , we observed that direct somatic application of rotenone, a mitochondria complex I targeting toxin, led to rapid (<4 h) and massive cell death and axonal degeneration, which was moderately but consistently reduced by BDV infection ( Supplementary Fig. 1 ). In contrast, axonal application of rotenone triggered axonal fragmentation, followed by a slow retrograde propagation of the degenerative process towards the cell body. Consequently, cell death was only evidenced at 24 and 48 h ( Supplementary Fig. 1 ), illustrating the advantages of this setup to model the dying-back pattern of neurodegeneration [21] . In this experimental paradigm, neuroprotection provided by BDV infection was still observed and even increased when compared with direct somatic injury. To specifically focus on axonal protection upon a localized insult by rotenone, we thus chose the 16 h time point, that is, before any signs of neuronal death. Observation of the axonal chambers revealed that treatment with rotenone for 16 h triggered extensive axonal degeneration ( Fig. 1a , compare upper and lower panels). Strikingly, BDV infection almost entirely abrogated rotenone-induced axonal fragmentation ( Fig. 1a,b ). A similar protection afforded by BDV infection against axonal fragmentation was observed after axonal treatment with mitochondria-penetrating peptide (MPP+), the active form of 1-methyl-4-phenyl-1,2,3,6-tetrahydropyridine (MPTP), another complex I targeting toxin that induces oxidative stress and which is widely used to model PD-like neurodegeneration in rodents and primates [22] ( Fig. 1c ). Since rotenone and MPP+ toxins were also reported to inhibit tubulin assembly by binding to tubulin, we used colchicine to inhibit microtubule polymerization and distinguish between both activities. Infection did not protect against colchicine-induced axonal fragmentation ( Fig. 1d ), showing that BDV specifically protects axons from complex I inhibition. 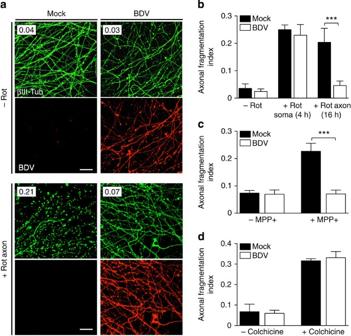Figure 1: BDV infection protects against rotenone-induced axonal fragmentation. (a) Representative example of confocal imaging of rotenone (Rot)-induced axonal fragmentation. Oriented neuronal cultures grown in microfluidic devices were mock- or BDV-infected (BDV) and treated (+Rot Axon) or not (−Rot) for 16 h with 1 μM rotenone added in the axonal chambers. The axonal network was stained for βIII-tubulin (Tub; green) to assess axonal morphology and for BDV nucleoprotein (red) to reveal infection. Inserts show the fragmentation indexes, calculated as described in the Methods section. (b) Quantification of axonal fragmentation, following 1 μM rotenone added either for 4 h directly in the somatic chamber (+Rot Soma) or for 16 h in the axonal chamber (+Rot Axon).n=4 independent experiments. (c,d) BDV infection protects from axonal fragmentation induced by toxins that target the mitochondria, but not against toxins that induce cytoskeleton damage. Quantification of axonal fragmentation in microfluidic-based oriented neuronal cultures, either mock or BDV infected, that were treated by axonal application during 16 h of (c) the respiratory complex I toxin MPP+ (10 μM) or (d) the tubulin polymerization inhibitor colchicine (10 μM).n=3 independent experiments. Scale bars, 10 μm. Data are represented as mean±s.d. ***P<0.001; Mann–Whitney test. Figure 1: BDV infection protects against rotenone-induced axonal fragmentation. ( a ) Representative example of confocal imaging of rotenone (Rot)-induced axonal fragmentation. Oriented neuronal cultures grown in microfluidic devices were mock- or BDV-infected (BDV) and treated (+Rot Axon) or not (−Rot) for 16 h with 1 μM rotenone added in the axonal chambers. The axonal network was stained for βIII-tubulin (Tub; green) to assess axonal morphology and for BDV nucleoprotein (red) to reveal infection. Inserts show the fragmentation indexes, calculated as described in the Methods section. ( b ) Quantification of axonal fragmentation, following 1 μM rotenone added either for 4 h directly in the somatic chamber (+Rot Soma) or for 16 h in the axonal chamber (+Rot Axon). n =4 independent experiments. ( c , d ) BDV infection protects from axonal fragmentation induced by toxins that target the mitochondria, but not against toxins that induce cytoskeleton damage. Quantification of axonal fragmentation in microfluidic-based oriented neuronal cultures, either mock or BDV infected, that were treated by axonal application during 16 h of ( c ) the respiratory complex I toxin MPP+ (10 μM) or ( d ) the tubulin polymerization inhibitor colchicine (10 μM). n =3 independent experiments. Scale bars, 10 μm. Data are represented as mean±s.d. *** P <0.001; Mann–Whitney test. Full size image BDV X protein mediates axonal protection To dissect the mechanism supporting the neuroprotective properties of BDV and to test the role of the X protein in axonal protection, we next compared the protective effects of a recombinant wild-type (wt) BDV (BDV-X wt ) with a recombinant BDV in which the X protein had been mutated to abrogate its mitochondrial localization (BDV-X A6A7 ) [10] . Consistent with the results shown above, infection with BDV-X wt strongly protected against rotenone-induced axonal fragmentation. In contrast, there was no protection with BDV-X A6A7 ( Fig. 2a ), establishing that the mitochondrial localization of the X protein is mandatory for axonal protection. To test whether the X protein could elicit neuroprotection by itself, we constructed lentiviral vectors (LVs) expressing green fluorescent protein (as a control) or various BDV proteins: the nucleoprotein (N), the phosphoprotein (P), the wt X protein (X wt ) or the X A6A7 mutant. Neurons grown in microfluidic devices were transduced with the different LV and axonal fragmentation was assayed 16 h after rotenone exposure of axons. Expression of X wt alone conferred similar level of axonal protection as infection with BDV ( Fig. 2b ). In addition, none of the other viral proteins induced similar protection. Here again, experiments using the LV-X A6A7 mutant established that the mitochondrial localization of the X protein was required for axonal protection. Confocal microscopy analysis of neurons transduced with LV-X wt and co-localization studies with mitochondrial Tom20 protein confirmed that the X protein indeed localizes to the mitochondria, even when expressed alone ( Fig. 2c,d ). 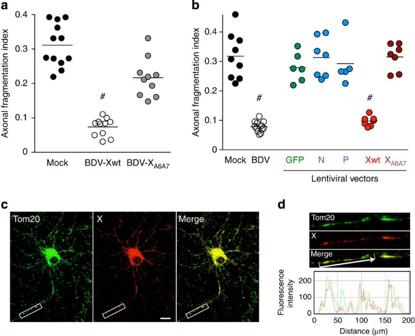Figure 2: BDV X protein mediates axonal protection even when expressed alone outside of the viral context. (a) Neurons grown in microfluidic devices were either mock treated or infected with wt recombinant BDV (BDV-Xwt) or recombinant BDV bearing mutations in the mitochondrial targeting sequence of X protein (BDV-XA6A7). Axonal fragmentation was quantified after treatment with 1 μM rotenone that was added in the axonal chamber for 16 h. (b) Analysis of axonal fragmentation in neurons transduced with LVs expressing independently each indicated protein (GFP or viral proteins N, P, X and mutant XA6A7) and treated with 1 μM rotenone in the axonal chamber for 16 h. Results obtained using mock- or BDV-infected neurons are also indicated in the figure for comparison. Each symbol ina,brefers to the fragmentation index calculated for one microfluidic culture and horizontal bars refer to the means.n=3 independent experiments. #P<10−4; Kruskal–Wallis test. (c,d) Analysis of X protein localization in mitochondria. Confocal imaging of neurons transduced with the LV expressing the X protein and stained for mitochondrial Tom20 (green) and BDV X (red). Right panel shows the merged image. (d) Enlarged picture of the white box shown inc. To better appreciate co-localization, below the pictures are plotted the intensity profiles of green and red fluorescent signals along the portion of the axon located above the white arrow. Scale bars, 10 μm (c) and 5 μm (d). Figure 2: BDV X protein mediates axonal protection even when expressed alone outside of the viral context. ( a ) Neurons grown in microfluidic devices were either mock treated or infected with wt recombinant BDV (BDV-X wt ) or recombinant BDV bearing mutations in the mitochondrial targeting sequence of X protein (BDV-X A6A7 ). Axonal fragmentation was quantified after treatment with 1 μM rotenone that was added in the axonal chamber for 16 h. ( b ) Analysis of axonal fragmentation in neurons transduced with LVs expressing independently each indicated protein (GFP or viral proteins N, P, X and mutant X A6A7 ) and treated with 1 μM rotenone in the axonal chamber for 16 h. Results obtained using mock- or BDV-infected neurons are also indicated in the figure for comparison. Each symbol in a , b refers to the fragmentation index calculated for one microfluidic culture and horizontal bars refer to the means. n= 3 independent experiments. # P <10 −4 ; Kruskal–Wallis test. ( c , d ) Analysis of X protein localization in mitochondria. Confocal imaging of neurons transduced with the LV expressing the X protein and stained for mitochondrial Tom20 (green) and BDV X (red). Right panel shows the merged image. ( d ) Enlarged picture of the white box shown in c . To better appreciate co-localization, below the pictures are plotted the intensity profiles of green and red fluorescent signals along the portion of the axon located above the white arrow. Scale bars, 10 μm ( c ) and 5 μm ( d ). Full size image BDV X protein preserves mitochondrial parameters Both rotenone and MPP+ block the formation of the electrochemical gradient across the inner mitochondrial membrane (ΔΨm). Using JC-1 as a ΔΨm indicator, we observed that BDV-X wt , but not the X A6A7 -mutated virus, prevented the time-dependent loss of ΔΨm in the axonal compartment of microfluidic neuronal cultures upon rotenone exposure, as evidenced by a decrease in the red/green fluorescence intensity ratios ( Fig. 3a,b ). Likewise, wt BDV also prevented rotenone-induced oxidative stress and burst of reactive oxygen species (ROS) production ( Fig. 3c,d ), whereas the X A6A7 -mutated virus had lost this property. The X protein is thus able to buffer mitochondrial dysfunctions triggered by complex I toxins and to preserve neurons from the resulting oxidative stress. 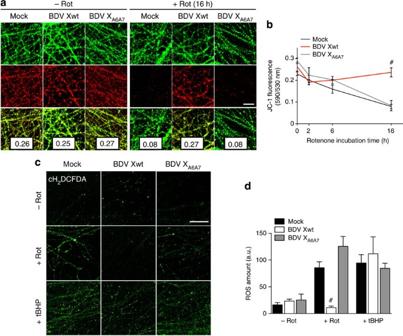Figure 3: BDV X protein protects from rotenone-induced oxidative stress. (a) Representative example of confocal analysis of axonal chambers of microfluidic devices loaded with the mitochondrial membrane potential (ΔΨm) indicator JC-1. Neurons were mock treated, infected with wt recombinant BDV (BDV-Xwt) or recombinant BDV bearing mutations in the mitochondrial targeting sequence of X protein (BDV-XA6A7). They were either left untreated (−Rot) or treated with 1 μm Rotenone (+Rot) added for 16 h in the axonal chamber. The JC-1 signals for JC-1 monomeric form (green fluorescence) and aggregated form (red fluorescence) are shown, together with the merged image (bottom panels). Inserts show the resulting red/green fluorescent ratio, whose drop upon rotenone exposure is indicative of mitochondrial depolarization. (b) Time-course analysis of ΔΨm (JC-1 fluorescence ratio) in the axonal chambers of microfluidic cultures of mock-, BDV-Xwt- and BDV-XA6A7-infected neurons after axonal treatment with 1 μM rotenone, showing that only BDV-Xwtstabilizes the mitochondrial membrane potential.n=3 independent experiments. (c) Representative example of confocal analysis of axonal chambers of microfluidic devices loaded with the reactive oxygen species (ROS) indicator H2-CFDA (green). Neurons were treated as described above. The positive control, that is, treatment with the ROS inducer tert-butyl hydroperoxide (tBHP) is also shown. (d) Quantification of ROS amounts (integrative fluorescence intensity measurements, expressed in arbitrary units (a.u.)).n=3 independent experiments. Scale bars, 5 μm (a,c). Data are represented as mean±s.d. #P<10−4; Kruskal–Wallis test. Figure 3: BDV X protein protects from rotenone-induced oxidative stress. ( a ) Representative example of confocal analysis of axonal chambers of microfluidic devices loaded with the mitochondrial membrane potential (ΔΨm) indicator JC-1. Neurons were mock treated, infected with wt recombinant BDV (BDV-X wt ) or recombinant BDV bearing mutations in the mitochondrial targeting sequence of X protein (BDV-X A6A7 ). They were either left untreated (−Rot) or treated with 1 μm Rotenone (+Rot) added for 16 h in the axonal chamber. The JC-1 signals for JC-1 monomeric form (green fluorescence) and aggregated form (red fluorescence) are shown, together with the merged image (bottom panels). Inserts show the resulting red/green fluorescent ratio, whose drop upon rotenone exposure is indicative of mitochondrial depolarization. ( b ) Time-course analysis of ΔΨm (JC-1 fluorescence ratio) in the axonal chambers of microfluidic cultures of mock-, BDV-X wt - and BDV-X A6A7 -infected neurons after axonal treatment with 1 μM rotenone, showing that only BDV-X wt stabilizes the mitochondrial membrane potential. n =3 independent experiments. ( c ) Representative example of confocal analysis of axonal chambers of microfluidic devices loaded with the reactive oxygen species (ROS) indicator H2-CFDA (green). Neurons were treated as described above. The positive control, that is, treatment with the ROS inducer tert-butyl hydroperoxide (tBHP) is also shown. ( d ) Quantification of ROS amounts (integrative fluorescence intensity measurements, expressed in arbitrary units (a.u.)). n =3 independent experiments. Scale bars, 5 μm ( a , c ). Data are represented as mean±s.d. # P <10 −4 ; Kruskal–Wallis test. Full size image The X protein reduces neuronal loss in MPTP-treated mice We then tested the neuroprotective properties of the X protein in vivo using the MPTP intoxication mouse model of PD [23] , [24] . LVs expressing either wt (LV-X wt ) or its non-mitochondrial mutant (LV-X A6A7 ) were introduced by stereotaxic injection in the substantia nigra pars compacta (SNpc), 2 weeks before MPTP intoxication. Immunofluorescence analysis using an anti-BDV X antibody was performed to confirm the distribution of the injected LV. Expression of the X protein was strong and was limited to the SNpc and in a restricted surrounding brain area ( Fig. 4a ). Moreover, confocal analysis of the co-localization with tyrosine hydroxylase (TH) revealed that a high proportion of TH-positive dopaminergic neurons in the SNpc also expressed the X protein ( Fig. 4b ). Three weeks after MPTP intoxication, the survival of nigrostriatal dopaminergic neurons was assayed by TH immunodetection in the striatum (axonal projections) or SNpc (cell bodies). As expected, intraperitoneal (i.p.) MPTP intoxication induced a bilateral lesion of the nigrostriatal pathway, which was evidenced by a decrease in striatal TH immunostaining ( Fig. 4c , compare upper and lower panels). The unilateral injection of LVs allowed us to evaluate the level of striatal protection for each mouse by comparison with the contralateral, non-injected side ( Fig. 4d ). This analysis was further complemented by the enumeration of surviving TH-positive neurons in the ipsilateral SNpc ( Fig. 4e,f ). MPTP-intoxicated mice that had been injected with LV-X A6A7 displayed a general loss of striatal fibres and loss of TH-positive neurons ( Fig. 4d,f ). In contrast, mice receiving LV-X wt were remarkably protected against MPTP toxicity, with a preservation of ipsilateral striatal fibres and an almost complete protection of ipsilateral TH-positive neurons in the SNpc ( Fig. 4d,f ). 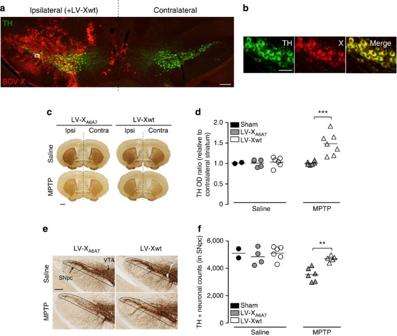Figure 4: The X protein protects against dopaminergic system degeneration in the MPTP mouse model of PD. (a) Immunofluorescence analysis upon ipsilateral (Ipsi) injection of LV-Xwtin the SNpc. Brains sections were stained with a BDV X antiserum (red) and tyrosine hydroxylase (TH; green) to reveal dopaminergic neurons. (b) Enlarged picture of the white box inais shown, allowing to appreciate the co-localization between staining for TH and X. (c) Representative photomicrographs of striatal sections immunostained for TH from saline- (top) or MPTP-intoxicated (bottom) mice, which were unilaterally injected (ipsilateral side) with LVs expressing wt (LV-Xwt) or mutated (LV-XA6A7) X proteins. (d) Quantification of striatal TH immunoreactivity (optical density, OD). For each mouse, data are expressed as the ratio of OD between the ipsilateral and the contralateral (Contra; non-injected) side, that is, any ratio >1 is indicative of neuroprotection. (e) Representative photomicrographs of midbrain sections immunostained for TH from the same animals shown above. The contours of the SNpc are delineated (dotted line) and the ventral tegmental area (VTA) above it, indicated. (f) Enumeration of surviving TH+dopaminergic neurons in the ipsilateral SNpc. The horizontal bars represent the mean number of TH+neurons. The investigator performing all quantifications was blinded to the treatment groups during the whole analysis process. Each symbol represents one animal.n=3 independent experiments. Scale bars, 100 μm (a,e), 15 μm (b) and 250 μm (c). **P<0.01; ***P<0.001; Mann–Whitney test. Figure 4: The X protein protects against dopaminergic system degeneration in the MPTP mouse model of PD. ( a ) Immunofluorescence analysis upon ipsilateral (Ipsi) injection of LV-X wt in the SNpc. Brains sections were stained with a BDV X antiserum (red) and tyrosine hydroxylase (TH; green) to reveal dopaminergic neurons. ( b ) Enlarged picture of the white box in a is shown, allowing to appreciate the co-localization between staining for TH and X. ( c ) Representative photomicrographs of striatal sections immunostained for TH from saline- (top) or MPTP-intoxicated (bottom) mice, which were unilaterally injected (ipsilateral side) with LVs expressing wt (LV-X wt ) or mutated (LV-X A6A7 ) X proteins. ( d ) Quantification of striatal TH immunoreactivity (optical density, OD). For each mouse, data are expressed as the ratio of OD between the ipsilateral and the contralateral (Contra; non-injected) side, that is, any ratio >1 is indicative of neuroprotection. ( e ) Representative photomicrographs of midbrain sections immunostained for TH from the same animals shown above. The contours of the SNpc are delineated (dotted line) and the ventral tegmental area (VTA) above it, indicated. ( f ) Enumeration of surviving TH + dopaminergic neurons in the ipsilateral SNpc. The horizontal bars represent the mean number of TH + neurons. The investigator performing all quantifications was blinded to the treatment groups during the whole analysis process. Each symbol represents one animal. n =3 independent experiments. Scale bars, 100 μm ( a , e ), 15 μm ( b ) and 250 μm ( c ). ** P <0.01; *** P <0.001; Mann–Whitney test. Full size image Identification of a neuroprotective X-derived peptide Despite these encouraging results, stereotaxic injection of neuroprotective compounds is invasive and cannot be envisioned as a convenient therapy [25] , [26] . Therefore, we asked whether small-cell-permeable peptides derived from the X protein could exhibit similar properties and be neuroprotective following systemic administration. In silico analysis of the X protein sequence did not reveal any homology with other viral or cellular proteins that would point to a particular domain involved in neuroprotection. Structure modelling ( Supplementary Fig. 2 ) predicts a highly disordered protein, except for a short N-terminal aliphatic alpha helix, that carries both nuclear and mitochondrial localization domains [27] . Thus, we synthesized three peptides covering the entire amino-acid sequence of the X protein to test each of them separately for neuroprotection ( Fig. 5a ). To ensure their targeting to mitochondria, we coupled these peptides with a MPP sequence (F-R-Cha-K-F-R-Cha-K, Cha, cyclohexylalanine), which was shown to allow both translocation of the plasma membrane and mitochondrial targeting with high specificity [28] . Since its original description, this MPP has been shown to allow the mitochondrial-specific delivery of a wide array of cargos, including fluorescent labels or drugs [29] , [30] , and its mitochondrial targeting properties have been observed by solid-state nuclear magnetic resonance [31] . We took advantage of the fact that the BDV X antibody also recognizes the PX3 peptide, corresponding to the C-terminal part of the X protein ( Fig. 5a ) to confirm that the MPP sequence indeed allowed its mitochondrial accumulation within 90 min of incubation in the medium of cultured neurons ( Fig. 5b ). The antibody, however, did not recognize the PX1 or PX2 peptides. We next assayed protection against rotenone-induced axonal fragmentation using our microfluidic neuronal culture model. Remarkably, peptide PX3 provided protection similar to that of full-length X protein ( Fig. 5c ). The other peptides did not exhibit any protection, suggesting that the neuroprotective property of the X protein resides entirely within its 29 amino-acid C-terminal sequence. 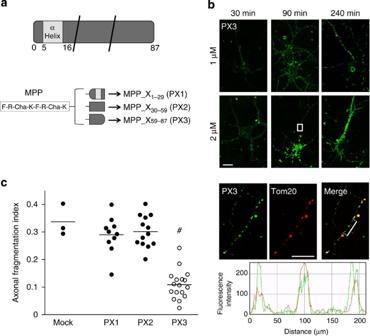Figure 5: A peptide covering the carboxy-terminal 29 amino acids of X protein displays axoprotective properties similar to that of the full-length protein. (a) Design of MPP-X peptides. Top, schematic representation of the X protein. Black bars indicate the limits of each peptide. Bottom, the same mitochondrial targeting, cell-permeable sequence (MPP) was added to each part of the X protein to obtain PX1, PX2 and PX3 peptides. The MPP sequence is shown on the left (Cha, cyclohexylalanine). (b) The PX3 peptide enters neurons and is targeted to mitochondria. Neurons were grown on glass coverslips for 9 days (5 × 104cells for each 12-mm-diameter coverslip). PX3 was added to the culture medium at different concentrations (1 or 2 μM) for various durations (30–240 min). Cells were processed for immunodetection of the peptide (using the anti-BDV X mouse polyclonal serum, green) and mitochondria network (anti-Tom20, red) and analysed by confocal microscopy. The lower panels show an enlarged portion of an axonal process. To better appreciate co-localization, below the pictures are plotted the intensity profiles of green and red fluorescent signals along the portion of the axon highlighted by the white line. (c) Analysis of rotenone-induced axonal fragmentation. Neurons grown in microfluidic devices were either mock treated or treated with the different peptides (2 μM). Axonal fragmentation was quantified after treatment with 1 μM rotenone that was added in the axonal chamber for 16 h. Each symbol refers to the fragmentation index calculated for one microfluidic culture and horizontal bars refer to the means.n=3 independent experiments. Scale bars, 10 μm (top panels), 5 μm (bottom panels). #P<10−4; Kruskal–Wallis test. Figure 5: A peptide covering the carboxy-terminal 29 amino acids of X protein displays axoprotective properties similar to that of the full-length protein. ( a ) Design of MPP-X peptides. Top, schematic representation of the X protein. Black bars indicate the limits of each peptide. Bottom, the same mitochondrial targeting, cell-permeable sequence (MPP) was added to each part of the X protein to obtain PX1, PX2 and PX3 peptides. The MPP sequence is shown on the left (Cha, cyclohexylalanine). ( b ) The PX3 peptide enters neurons and is targeted to mitochondria. Neurons were grown on glass coverslips for 9 days (5 × 10 4 cells for each 12-mm-diameter coverslip). PX3 was added to the culture medium at different concentrations (1 or 2 μM) for various durations (30–240 min). Cells were processed for immunodetection of the peptide (using the anti-BDV X mouse polyclonal serum, green) and mitochondria network (anti-Tom20, red) and analysed by confocal microscopy. The lower panels show an enlarged portion of an axonal process. To better appreciate co-localization, below the pictures are plotted the intensity profiles of green and red fluorescent signals along the portion of the axon highlighted by the white line. ( c ) Analysis of rotenone-induced axonal fragmentation. Neurons grown in microfluidic devices were either mock treated or treated with the different peptides (2 μM). Axonal fragmentation was quantified after treatment with 1 μM rotenone that was added in the axonal chamber for 16 h. Each symbol refers to the fragmentation index calculated for one microfluidic culture and horizontal bars refer to the means. n =3 independent experiments. Scale bars, 10 μm (top panels), 5 μm (bottom panels). # P <10 −4 ; Kruskal–Wallis test. Full size image Intranasal administration of PX3 is neuroprotective in vivo We next examined whether PX3 could be protective in the MPTP mouse model of PD, similarly to our findings with the full-length X protein. We first assessed neuroprotection upon direct delivery of the peptides in the CNS by intra-cerebroventricular (ICV) injection. When compared with lesions observed in MPTP-intoxicated mice that had been injected with the PX2 peptide, we observed that ICV injection of PX3 peptide led to 40% and 53% protection against MPTP-induced loss of striatal TH fibres and SNpc TH-positive neurons, respectively, ( Supplementary Fig. 3 ). In order to explore a more convenient systemic route of administration, we then performed intranasal instillations of the peptide. Indeed, the intranasal route is known to bypass the blood–brain barrier through olfactory- and trigeminal-associated extracellular pathways, allowing entry of agents to the CNS, as shown for insulin-like growth factor-1 (ref. 32 ). Moreover, intranasal intoxication by MPTP constitutes a new route of toxin delivery in the brain that mimics environmental exposure to neurotoxins [33] , further demonstrating the ability of chemicals to get from the olfactory bulb to the nigrostriatal pathway, as shown recently using Matrix-assisted laser desorption/ionization (MALDI) mass spectrometry imaging [34] . To determine whether delivery of PX3 peptide into the brain could also be achieved by intranasal administration, we performed experiments using radiolabelled PX3, and analysed its distribution in several peripheral organs and in the CNS ( Table 1 ). Following intranasal administration, we detected PX3 in the periphery, notably in the lung, intestine and kidney, probably resulting from peptide spill over to the respiratory and digestive tracts during intranasal administration. As anticipated, the highest levels in the CNS were evidenced in the olfactory bulb. In addition, PX3 was detected in all sites of the brain and spinal cord, with a marked preference for the striatum and mesencephalon, demonstrating that the PX3 peptide could indeed bypass the blood–brain barrier and target the brain region of interest for us, that is, the nigrostriatal pathway. We next challenged the effect of PX3 on MPTP-induced neurodegeneration. Since dopaminergic neuronal insult occurs mainly within the first 4 days after acute MPTP intoxication [23] , we intranasally delivered the peptides daily, one day before i.p. MPTP intoxication and during the following 4 days. No adverse reaction or clinical signs were noted with the daily intranasal application of PX2 or PX3 peptides. Histological analysis of the brains 3 weeks after MPTP intoxication revealed that mice of the control group, which had received the non-protective PX2 peptide, displayed a marked loss of TH-positive neurons ( Fig. 6a,b ) and striatal dopaminergic fibres ( Fig. 6c,d ). Strikingly, when mice had received the PX3 peptide, the lesions were reduced by 40%, both in the striatum and the SNpc ( Fig. 6b,d ). Table 1 Tissue concentrations of [ 125 I]-labelled PX3 peptide following intranasal administration. 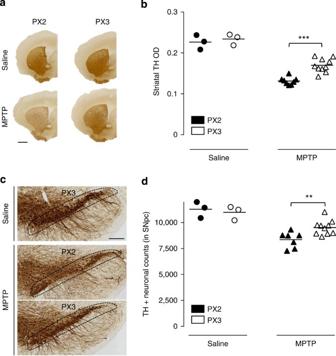Figure 6: Intranasal administration of PX3 protects neurons from neurodegeneration in MPTP-treated mice. (a) Representative photomicrographs of striatal TH immunostaining from saline-treated or MPTP-intoxicated mice that had received intranasal administration of PX2 or PX3 peptides. (b) Quantification of striatal TH immunoreactivity (optical density, OD). (c) Representative photomicrographs of mesencephalic sections immunostained for TH from the same animals. The contours of the SNpc are delineated (dotted line) (d) Enumeration of surviving TH+ dopaminergic neurons in the whole SNpc. The investigator performing the quantifications was blinded to the treatment groups during the whole analysis process. Each symbol represents one animal.n=3 independent experiments. Scale bars 100 μm (a), 250 μm (c). **P<0.01; ***P<0.001; Mann–Whitney test. Full size table Figure 6: Intranasal administration of PX3 protects neurons from neurodegeneration in MPTP-treated mice. ( a ) Representative photomicrographs of striatal TH immunostaining from saline-treated or MPTP-intoxicated mice that had received intranasal administration of PX2 or PX3 peptides. ( b ) Quantification of striatal TH immunoreactivity (optical density, OD). ( c ) Representative photomicrographs of mesencephalic sections immunostained for TH from the same animals. The contours of the SNpc are delineated (dotted line) ( d ) Enumeration of surviving TH+ dopaminergic neurons in the whole SNpc. The investigator performing the quantifications was blinded to the treatment groups during the whole analysis process. Each symbol represents one animal. n =3 independent experiments. Scale bars 100 μm ( a ), 250 μm ( c ). ** P <0.01; *** P <0.001; Mann–Whitney test. Full size image Both X and PX3 induce mitochondrial elongation The underlying mechanism of protection conferred by the X protein and PX3 against mitochondrial poisoning was investigated further. Confocal microscopy analysis revealed that neurons expressing the X protein exhibited a marked increase in mitochondrial elongation ( Fig. 7a ). The same analysis was repeated in neurons expressing X A6A7 or treated with the PX3 peptide, both under basal conditions and after rotenone-induced oxidative stress. Quantitative analysis of mitochondria size distribution confirmed that the expression of X or PX3, but not mutant X A6A7 , resulted in a more filamentous network under basal conditions, with a 60% decrease of short, fragmented mitochondria (<2 μm) and a four- to fivefold increase in long mitochondria (>8 μm; Fig. 7b ). Importantly, when a similar analysis was undertaken after rotenone exposure, we observed that both the X protein and the PX3 peptide significantly reduced rotenone-induced mitochondrial fission ( Fig. 7c ), thus preserving the presence of elongated mitochondria. 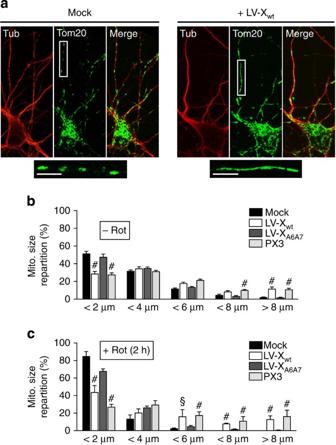Figure 7: The X protein and PX3 trigger filamentation of the mitochondrial network both under basal conditions and after oxidative stress. (a) Representative example of a confocal analysis of non-transduced neurons (Mock) and of neurons transduced with the LV expressing X (LV-Xwt). Neurons were stained for neuronal βIII-tubulin (Tub; red) and the mitochondrial marker Tom20 (green). Lower panels show a higher magnification of the boxed area to illustrate the impact of the X protein on mitochondrial elongation. (b,c) Analysis of mitochondria (Mito.) size distribution in control neurons (Mock), in neurons transduced with LVs expressing either Xwt(LV-X) or XA6A7(LV-XA6A7), as well as in neurons treated with PX3. Analysis was performed (b) without treatment (−Rot) or (c) after rotenone (Rot) treatment (10 nM) for 2 h (+Rot). Data were obtained from at least 15 neurons in each group and for each experiment, and are expressed as mean±s.d.n=3 independent experiments. The investigator performing the quantification was blinded to the treatment groups during the whole analysis process. Scale bars, 5 μm. #P<10−4; §P<10−3; Kruskal–Wallis test. Figure 7: The X protein and PX3 trigger filamentation of the mitochondrial network both under basal conditions and after oxidative stress. ( a ) Representative example of a confocal analysis of non-transduced neurons (Mock) and of neurons transduced with the LV expressing X (LV-Xwt). Neurons were stained for neuronal βIII-tubulin (Tub; red) and the mitochondrial marker Tom20 (green). Lower panels show a higher magnification of the boxed area to illustrate the impact of the X protein on mitochondrial elongation. ( b , c ) Analysis of mitochondria (Mito.) size distribution in control neurons (Mock), in neurons transduced with LVs expressing either X wt (LV-X) or X A6A7 (LV-X A6A7 ), as well as in neurons treated with PX3. Analysis was performed ( b ) without treatment (−Rot) or ( c ) after rotenone (Rot) treatment (10 nM) for 2 h (+Rot). Data were obtained from at least 15 neurons in each group and for each experiment, and are expressed as mean±s.d. n =3 independent experiments. The investigator performing the quantification was blinded to the treatment groups during the whole analysis process. Scale bars, 5 μm. # P <10 −4 ; § P <10 −3 ; Kruskal–Wallis test. Full size image Both X and PX3 reduce Drp1 S616 phosphorylation We next assessed whether the enhanced mitochondrial elongation stimulated by X or PX3 could result from changes in the expression and/or activation of proteins involved in mitochondrial fission or fusion processes. We did not find any significant difference in the expression levels of the fusion proteins Optical Atrophy 1 and mitofusins 1 and 2 or in the fission protein Fis1 (Data not shown). We next focused on the dynamin-related protein 1 (Drp1) because of its central role in the regulation of mitochondrial morphology in neurons [2] . Confocal microscopy analyses suggested that expression of total Drp 1 was not affected by the expression of X wt ( Fig. 8a ). Strikingly, however, levels of Drp1 phosphorylation at serine 616 residue (Drp1 S616 ), a phosphorylation site known to regulate mitochondrial fission [35] , were strongly reduced in X-expressing or PX3-treated neurons, but not with the non-mitochondrial X A6A7 mutant ( Fig. 8b,c ). Following treatment with rotenone, we observed increased Drp1 S616 phosphorylation associated with enhanced mitochondrial fission. Here again, the rotenone-induced increased Drp1 S616 phosphorylation was selectively reduced by X expression or PX3 treatment. 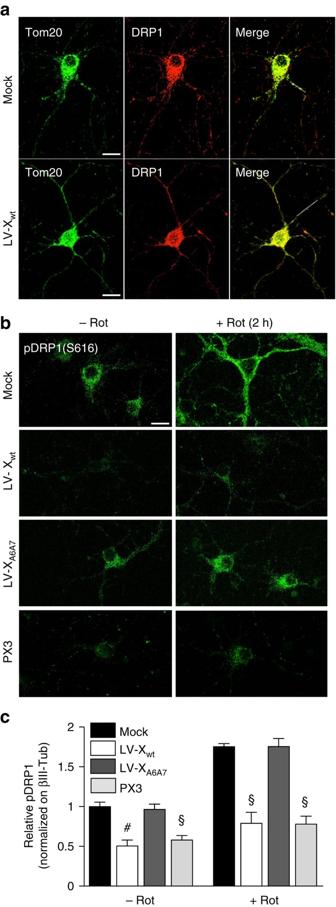Figure 8: The X protein and PX3 block Drp1S616phosphorylation both under basal conditions and after oxidative stress. (a) Representative example of a confocal analysis of immunostaining for the mitochondrial marker Tom20 (green) and total Drp1 (red) in control neurons (Mock) or in neurons transduced with the LV expressing Xwt(LV-Xwt). Merged images are show on the right. Similar results were observed for at least 20 cells for each experiment.n=4 independent experiments. (b) Confocal analysis of immunostaining for phospho-Drp1S616. Analysis was performed under basal conditions (−Rot) or after rotenone (Rot) treatment (10 nM) for 2 h (+Rot 2 h). (c) Quantitative analysis of phospho-Drp1S616, showing that Xwtprotein or PX3 block rotenone-induced Drp1S616phosphorylation. Scale bars, 10 μm. Each measure was obtained by measuring the integrative intensity of three randomly chosen fields, normalized on total βIII-tubulin (Tub) staining of the same area, using ImageJ software and fixed thresholds. Data are expressed as mean±s.d.n=6 independent experiments. #P<10−4; §P<10−3; Kruskal–Wallis test. Figure 8: The X protein and PX3 block Drp1 S616 phosphorylation both under basal conditions and after oxidative stress. ( a ) Representative example of a confocal analysis of immunostaining for the mitochondrial marker Tom20 (green) and total Drp1 (red) in control neurons (Mock) or in neurons transduced with the LV expressing X wt (LV-Xwt). Merged images are show on the right. Similar results were observed for at least 20 cells for each experiment. n =4 independent experiments. ( b ) Confocal analysis of immunostaining for phospho-Drp1 S616 . Analysis was performed under basal conditions (−Rot) or after rotenone (Rot) treatment (10 nM) for 2 h (+Rot 2 h). ( c ) Quantitative analysis of phospho-Drp1 S616 , showing that X wt protein or PX3 block rotenone-induced Drp1 S616 phosphorylation. Scale bars, 10 μm. Each measure was obtained by measuring the integrative intensity of three randomly chosen fields, normalized on total βIII-tubulin (Tub) staining of the same area, using ImageJ software and fixed thresholds. Data are expressed as mean±s.d. n =6 independent experiments. # P <10 −4 ; § P <10 −3 ; Kruskal–Wallis test. Full size image During chronic neurodegenerative diseases such as PD or Alzheimer’s diseases, neuronal loss usually proceeds through a protracted dying-back pattern in which dysfunction of nerve endings and axonal demise long precedes neuronal cell body destruction [36] . Thus, protecting nerve endings from degeneration appears an important goal in order to achieve efficient neuroprotection in the brain. Although several approaches have been undertaken to specifically buffer axonal stress, such as treating with neurotrophins or increasing antioxidant defences [37] , they have yielded unequal success because of the dual role of these molecules in both axonal damage and signalling. Here, our data show that the X protein promotes a specific axoprotective effect and significant neuroprotection in a mouse model of PD, notably by modulating mitochondrial dynamics. Our results made a critical distinction between protection against somatic cell death, which was only modest in vitro , and the strong axonal protection conferred by the X protein that translated thereafter in efficient protection in the animal model. Our initial observations were facilitated by the use of oriented cultures grown in microfluidic chambers. With this setting, the retrograde propagation of the degenerative process towards the cell body of neurons upon axonal exposure to rotenone is delayed, presumably because it is buffered by the anterograde transport of undamaged material, thus deferring somatic degeneration [38] , [39] . The differences between somatic versus axonal protection conferred by the X protein or the PX3 peptide are likely owing to the fact that the molecular mechanisms involved in somatic and axonal degeneration differ significantly [21] , [40] , [41] . Axons are enriched in anti-apoptotic signalling molecules, such as the NAD + signalling pathway, which controls axonal fate after local insults [42] , [43] . Similar to the findings reported here, NAD + protects axons, but not the soma, upon global and/or local insults [19] , [44] . Mitochondrial network dynamics plays a major role in mitochondria quality control and has emerged as a central actor in neurodegeneration [45] , [46] , [47] . Generally, the mitochondrial network becomes fragmented in response to stress, in order to facilitate mitophagy of damaged mitochondria, whereas a filamentous network ensures a better response to oxidative stress, both through dilution of stress molecules and compensatory mechanisms [48] , [49] . We observed that mitochondrial elongation stimulated by the X protein or the PX3 peptide was accompanied by reduced Drp1 S616 phosphorylation. Since Drp1 phosphorylation occurs in the cytoplasm and it is recruited at the outer mitochondrial membrane for fission, it is puzzling that only the mitochondrial-targeted X, as opposed to the mutant protein, was able to decrease Drp1 S616 phosphorylation. In addition, co-immunoprecipitation experiments did not reveal any interaction between Drp1 and X proteins (data not shown). We therefore postulate that the X protein may induce modifications of the activity of cellular kinases through mitochondria–cytoplasm cross talk. Phosphorylation of Drp1 S616 is mediated by multiple kinases, including CDK1 during mitosis [35] , ERK1/2 under high glucose conditions [50] or PKCδ during hypertension [51] . Interestingly, very recent results showed that CDK5 is involved in the phosphorylation of Drp1 S616 in cultured rat neurons [52] . Alternatively, the impact of the X protein on Drp1 S616 phosphorylation may be secondary to its action on the respiratory chain by buffering ROS production and preserving membrane potential, which also are likely to impact on mitochondrial fission. Thus, a full understanding of the molecular mechanisms whereby the X protein acts on this balance of kinase activities and on Drp1 S616 phosphorylation clearly requires further research. Importantly, we showed that the C-terminal end of the X protein, enclosed within PX3, was able to protect against neurodegeneration in vitro and in vivo at levels comparable to the full-length protein. We cannot however totally exclude the possibility that other parts of the protein may also be effective. Indeed, we could not formally show that PX1 and PX2 peptides were actually delivered to cells because of a lack of reagents to detect them. However, the well-established flexibility and versatility of the MPP transporter also present in PX1 and PX2 suggest that it most likely the case. Notwithstanding such possibility, the intranasal administration of PX3 markedly reduced axonal damage and neuronal loss in the MPP mouse model of PD. This relatively minimally invasive method holds great promise for future therapeutics. Often, efficient drug candidates in vitro were found to exert little impact on the outcome of neurodegenerative diseases in animal models or in clinical trials because of their inability to be adequately delivered across the blood–brain barrier. The identification of anatomical routes connecting the nasal passages, the brainstem and the spinal cord has paved the way for new treatment paradigms of CNS diseases by intranasal administration, using drug candidates such as peptides [53] or liposome-encapsulated molecules [54] . Neurodegenerative diseases represent a considerable human, societal and economic burden, which is continually growing with the ageing of populations worldwide. Many emerging experimental neuroprotection strategies aimed at controlling apoptosis act at the level of post-mitochondrial effectors, such as caspase inhibition or by preventing mitochondrial membrane permeabilization [55] . Thus, there is a clear window of opportunity for targeting upstream phenomena such as the regulation of mitochondrial homeostasis and oxidative stress injury, especially when considering the growing evidence of the role of mitochondrial dynamics in neurodegeneration [56] . Our findings show that the X protein and the PX3 peptide target a major culprit in neurodegeneration. These virus-derived peptides therefore define a new class of neuroprotective agents with great potential for the treatment of patients suffering from PD. Moreover, the effects of PX3 peptide may be therapeutically beneficial in other diseases where impaired mitochondrial dynamics or function is central to disease pathogenesis. Animals Eight-week-old male C57BL/6 mice (Charles River Laboratories) were provided with food and water ad libitum and maintained in a temperature-controlled environment in a 12/12 h light–dark cycle. Animal handling and care was performed in accordance with the European Union Council Directive 86/609/EEC, and experiments were performed following the French national chart for ethics of animal experiments (articles R 214- 87 to 90 of the ‘Code rural’). Our protocol received approval from the local committee on the ethics of animal experiments (permit number: 13CB-U1043 DD-11), and all efforts were made to minimize animal numbers and suffering. Cells and virus strains HEK-293T cells (ATCC CRL-3216) were passaged 1:10 twice a week in DMEM (Gibco) supplemented with 10% fetal calf serum (Gibco), 2 mM L -glutamine (GE Healthcare) and 0.2 mg ml −1 geneticin (Gibco). Cell-released virus stocks were prepared as described [57] , [58] using Vero cells (ATCC CCL-81) infected with either BDV (Giessen strain He/80) or recombinant viruses expressing wt or mutated X (rBDV-LRD-Xwt and rBDV-LRD-X A6A7 , a kind gift from U. Schneider, Freiburg University, Germany). Timed pregnant Sprague–Dawley female rats were purchased from Janvier Labs. Primary cortical neurons were prepared from rat embryos at gestational day 17. After dissection, cortex tissue was dissociated by a 15-min incubation at 37 °C in PBS containing 10 U ml −1 Papain (Worthington) followed by a gentle dissociation in PBS containing 1.5 mg ml −1 bovine serum albumin (BSA) and 1.5 mg ml −1 trypsin inhibitor (from chicken egg, Sigma-Aldrich). After centrifugation through a 4% BSA cushion, neurons were plated on culture dishes coated with 0.5 mg ml −1 poly- DL -ornithine (overnight, Sigma-Aldrich) and 5 μg ml −1 laminin (2 h, Roche). Neuronal cultures were maintained in complete neuronal culture medium composed of serum-free Neurobasal (Gibco) supplemented with 2 mM L -glutamine, 100 μg ml −1 penicillin/streptomycin (Gibco) and 2% B-27 supplement (Gibco). Microfluidic culture chambers and neuronal culture setting Microfluidic chips were prepared as described elsewhere [18] , [19] . In brief, culture chambers were moulded with polydimethylsiloxane (Sylgard 184, Dow Corning; 9:1 ratio with curing agent), which was poured into resin SU-8 silicon masters having a complementary positive relief pattern of the cell culture compartments and microchannels. The resulting elastomeric polymer prints were detached and reservoirs were created using a biopsy puncher. After cleaning with isopropanol and air-drying, polymer prints and glass coverslips were treated for 1 min with an air plasma generator. Both elements were then bonded together, hydrated with sterile water, sterilized under ultraviolet for 15 min and coated with poly- DL -ornithine and laminin. Primary neuronal cultures prepared as described above were adjusted to a final concentration of 5 × 10 7 cells per ml and cell suspensions were seeded in the somatic chambers by introducing 3 μl in the upper reservoir. After 1 or 2 min, when neurons had attached to the substrate, reservoirs were filled with complete neuronal culture medium. A 10-μl differential medium volume was maintained between the somatic and axonal chambers to ensure a permanent hydrostatic flux. Neurons were infected with the different cell-free BDV strains described above 1 day after plating or they were transduced with LVs 3 days after plating. Construction and production of LVs The genes encoding BDV N (nucleoprotein), P (phosphoprotein), X, mutated X A6A7 (ref. 10 ) or green fluorescent protein were amplified by PCR and cloned into the pTrip LV backbone (kind gift from Dr P. Charneau, Pasteur Institute, Paris) using BamHI and XhoI restriction sites, downstream the constitutive cytomegalovirus enhancer/chicken β-actin (CAG) promoter. To produce the LVs, 10 T150 flasks plated with 1.2 × 10 7 HEK-293T cells each were transfected with packaging plasmids psPAX2 and pMD2.G (both from Addgene), and pTrip expressing the different genes (respectively 14.6, 7.9 and 22.5 μg of endotoxin-free prepared plasmids mixed with 100 μl of GeneJuice (Merck) for each T150). Culture medium was removed the next day and replaced by warm OptiMEM (Gibco). Supernatants were collected 48 and 72 h post transfection, cleared by low-speed centrifugation and filtered using a 0.45-μm filter, and lentiviral particles were purified by ultracentrifugation through a 20% sucrose cushion (25,000 r.p.m., 2 h, 4 °C; SW32Ti rotor, Beckman Coulter). Ice-cold PBS was added to each centrifugation tube and lentivector-containing pellets were let to swell under gentle agitation overnight at 4 °C, before being recovered, aliquoted and stored at −80 °C. Lentivector titres were determined by counting foci 72 h after transduction of HEK-293T cells with serial dilutions. In all our experiments, titres varied from 8 × 10 8 to 3 × 10 9 TUs per millilitre, and LVs were used at a multiplicity of transduction of 5 (TUs of vector for each cell) for in vitro neuronal transductions. Induction of axonal or somatic oxidative stress Twelve-day-old neuronal cultures were subjected to oxidative stress by adding the respiratory chain complex I inhibitors rotenone (1 μM, diluted in DMEM containing 1 g l −1 glucose (Invitrogen), supplemented with 2 mM glutamine+1% penicillin/streptomycin+2% B-27+1% N2 supplements (Invitrogen)) or MPP+ (1-methyl-4-phenylpyridinium ion, 10 μM in complete neuronal culture medium). The microtubule inhibitor colchicine (10 μM, complete neuronal culture medium) was used as a non-mitochondrial stress control. Toxins were added in the somatic or axonal chambers for somatic or axonal stress, respectively. Immunofluorescence and imaging in microfluidic chambers Neurons in the microfluidic cultures were fixed for 40 min at room temperature with PBS containing 4% paraformaldehyde (PFA), permeabilized using PBS+0.1% Triton X-100 during 20 min, rinsed with PBS and blocked for 2 h with PBS+2.5% normal goat serum+3% BSA (blocking buffer). Incubation for at least 2 h at room temperature with primary antibodies diluted in blocking buffer was followed, after extensive washes in PBS, by 1 h incubation at room temperature with fluorescently conjugated secondary antibodies diluted in PBS. For TOPRO3 staining, somatic chambers were incubated with TOPRO3 (1:1,000 in PBS; Invitrogen) for 10 min and then rinsed twice in PBS. All times for incubations and washes were reduced by 50% for neurons grown in standard coverslips. Fluorescence-based analyses and measurements were performed on either Zeiss LSM-510 or Zeiss LSM-710 inverted confocal microscopes with a × 40 objective ( × 63 objective for the analysis of mitochondrial network morphology and quantification of phospho-Drp1 S616 immunoreactivity). Immunofluorescence analyses of Drp1 were performed using anti-phospho-Drp1 S616 (Cell Signaling Technologies, diluted 1:1,000). Quantification of fluorescence intensities was performed using the threshold-based fluorescence quantification module of ImageJ software. All data were normalized on βIII-tubulin staining. Analysis of axonal fragmentation The analysis of axonal degeneration was adapted from the image segmentation method described by Kilinc et al. [18] The analysis was performed both by phase contrast observation and after immunostaining of axonal βIII-tubulin (Sigma-Aldrich, diluted 1:1,000). Intact axons present linear phase contrast morphology and a homogeneous tubulin staining delineating the axon shaft, whereas blebbed or severed axons exhibit a fragmented morphology and punctate tubulin network. For each microfluidic culture, the total βIII-tubulin staining area was measured on four randomly chosen fields in low-density axonal areas of the axonal chamber (MetaMorph software analysis, fixed thresholds). Low-density axonal areas were preferred for image analysis because an extensive overlap of neuronal processes would complicate the definitive identification of individual axons. Then, the number of tubulin spots of fragmented axons was manually counted (Imaris software, Spot counting for ‘clicking’ records), and the ratio between the number of spots and the total staining area was defined as a fragmentation index. To control for infection or transduction efficiencies, immunostaining for BDV antigens (using homemade rabbit antisera raised against N, P or X proteins) were performed together with βIII-tubulin. To ensure that the hydrostatic flux had indeed prevented drugs from diffusing back to the somas through the channels, TOPRO3 (Invitrogen) staining was performed in somatic chambers and nuclear integrity was checked for each culture. The observation of >25% fragmented/dead nuclei in control or axonal-damaged cultures was an exclusion criterion. Synthesis and use of X-derived peptides Peptides covering the N-terminal (PX1, aa 1–29), middle (PX2, aa 30–59) or C-terminal (PX3, aa 59–87) parts of BDV X protein (GenBank: ABW81015.1) coupled to the MPP sequence were synthesized to >95% ( in vitro studies) or >99% ( in vivo studies) purity (Génosphère Biotechnologies). For in vitro experiments, neurons were grown for 12 days before replacing the medium by fresh complete neuronal culture medium containing 2 μM of the peptides. The cultures were maintained for 90 min at 37 °C, 5% CO 2 before any treatment or analysis to ensure peptide penetration into neuronal mitochondria. For ICV delivery, peptides were injected as described below. For intranasal peptide delivery, each mouse was cradled in a vertical position and the peptide solution (1 mg ml −1 solution in saline: H 2 O+0.9% NaCl) was applied using a pipette and tip. A quantity of 10 μl drops were placed onto the mice nostrils and then absorbed by the mouse daily from the day before to the third day after MPTP intoxication. Determination of PX3 content in organs and brain structures Radioiodination of PX3 peptide (>99% pure) was performed with [ 125 I] using a Bolton–Hunter procedure (Custom Iodination service, PerkinElmer, Billerica, USA). The [ 125 I]-labelled PX3 (initial specific activity: 2,200 Ci mmol −1 ) was further purified by high-pressure liquid chromatography to eliminate remaining unbound iodine. On the day of each experiment, the activity (c.p.m. per microlitre) of the labelled peptide was determined by replicate sampling and counting using a 1,450 Microbeta Trilux counter (PerkinElmer). Intranasal delivery of the PX3 peptide was performed as described above. One hour after the last peptide administration, a detailed necropsy was performed on each animal, exercising care to avoid cross-contamination of tissues. After gross dissection of several peripheral organs, discrete brain areas were microdissected under magnifying glasses with a razor blade and forceps (Fine Science Tools) by using a micropunch technique. Control animals received the same volume of saline intranasally and were processed similarly. The weight of each dissected tissue was determined with a precision balance before gamma counting. Tissue concentrations (picomoles per gram of tissue) were calculated using the specific activity of the administered [ 125 I]-PX3, after subtraction of background radioactivity, corresponding to results of the counting of each corresponding organ (or brain area) from control animals. Stereotaxic surgery Unilateral stereotaxic injections of LVs were performed into the SNpc of 8-week-old mice at the following coordinates: Anterior-Posterior (AP) −2.6 mm relative to Bregma, Medial-Lateral (ML) +1.2 mm and Dorsal-Ventral (DV) −4.4 mm from the dura. Each mouse was injected with 1.10 6 TUs of vectors in a volume of 1 μl at the flow rate of 0.1 μl min −1 using a 10-μl microsyringe (Hamilton). Mice were rested post operation for 2 weeks before MPTP intoxication. For ICV delivery of peptides, cannulas (Phymep) were stereotaxically implanted into the lateral ventricle through a hole drilled in the skull at the following coordinates: AP 0.0 mm relative to Bregma, ML +1.0 mm, and DV −2.0 mm from skull. Dental cement was used to fix the cannula guide to the skull (polycarboxylate, Sigma-Aldrich) and to prevent occlusion. Mice were rested post operation for 2 weeks before peptide delivery and subsequent MPTP intoxication. Peptide was injected through the cannulas by fixation of an injector (Phymep) connected to a peristaltic pump, the day before and every day for 3 days after intoxication (2 nmol in 2 μl for each injection, injection rate: 0.5 μl min −1 ). MPTP intoxication and tissue processing For MPTP intoxication, mice were injected i.p. four times at 2 h intervals with either 18.5 mg kg −1 MPTP-HCl (as free base, Sigma-Aldrich, ref. no. M0896) or a corresponding volume of 0.9% NaCl solution. Mice were kept for 3 weeks to ensure lesion stabilization before killing. Mice were anaesthetized with a mixture of ketamine hydrochloride (100 mg kg −1 , i.p.) and xylazine (15 mg kg −1 , i.p.) dissolved in isotonic saline sterile solution or with sodium pentobarbital (150 mg kg −1 , i.p. ), and transcardiacally perfused at a flow rate of 5 ml min −1 with PBS (20 ml) followed by ice-cold 4% PFA (100 ml). After extraction from the skull, brains were further post fixed overnight in fresh 4% PFA solution and cryoprotected with 30% sucrose in phosphate buffer. Brains were then frozen by immersion in −30 °C isopentane and kept at −80 °C until further processing. Series of striatal and mesencephalic coronal sections (20-μm thick) were collected using a freezing microtome (Thermo Scientific) and stored in PBS containing 0.3% sodium azide. Immunohistochemistry and image analysis For immunohistochemical staining, free-floating brain sections were first quenched for 5 min in 20% (v/v) methanol and 1% (v/v) hydrogen peroxide diluted in PBS, then blocked for 30 min in a 4% solution of BSA diluted in PBS-0.3% Triton X-100 and incubated overnight at 4 °C with a primary antibody directed against TH (1:500 dilution, US Biological). After extensive washing in PBS, the sections were incubated for 1 h with biotinylated secondary antibody (1:250 dilution; Vector Laboratories). Staining was visualized by the ABC method (Vector Laboratories) with 3,3'-diaminobenzidine as the peroxidase substrate. TH-positive neurons were quantified stereologically on regularly spaced sections covering the whole SNpc. The SNpc was delineated [59] and TH-positive cell bodies were counted by bright-field microscopy, using a Leitz microscope equipped with image analysis software (Mercator, ExploraNova, La Rochelle, France). Of note, the analysis was focused on the SNpc, since ventral tegmental area dopaminergic neurons are much less sensitive to MPTP [59] . Striatal TH optic densitometry was quantified using the MCID software (MCID analysis 7.0). Staining background measured in the cerebral cortex was subtracted from striatal density measurements. The investigator performing the quantification was blinded to the treatment groups during the whole analysis process. Analysis of mitochondrial membrane potential Axons were stained with JC-1 dye (2 μM in PBS; Life Technologies) following recommendations of the manufacturer. In brief, JC-1 was added to the culture medium for 45 min at 37 °C, 5% CO 2 , washed twice with PBS and analysed by confocal microscopy using 488 nm excitation together with 530 and 585 nm band-pass emission filters, while maintaining the cells at 37 °C and 5% CO 2 . Total fluorescence intensity was measured for each emission band pass with fixed thresholds, and ratios between ‘red’ (585 nm, aggregated JC-1) and ‘green’ (530 nm, monomeric JC-1) were determined for each culture (means of four randomly chosen fields for each microfluidic culture). Measurement of ROS production The culture medium was removed from the axonal or somatic chambers and replaced by pre-warmed PBS containing carboxy-2′,7′-dichlorodihydrofluorescein diacetate (5 μM in PBS; Life Technologies) for 45 min at 37 °C, 5% CO 2 . After two washes in PBS, cultures were returned to warm culture medium for 30 min. Cells were fixed and the integrative fluorescence was measured on three randomly chosen fields for each axonal chamber. Tert -butyl hydroperoxide (Life Technologies) was used as a positive control of ROS detection. ROS amounts were detected by fluorescence (excitation/emission: 495/529 nm) and quantified by measuring integrative emission signal intensities for each culture (mean of four randomly chosen fields for each microfluidic culture, using Zeiss LSM-510 confocal). Analysis of mitochondrial network morphology Neurons were grown for 9 days at low density on 12–mm–diameter glass coverslips placed in 24-well plates (5 × 10 4 cells in each well). Transduction with LVs was performed on day 3, whereas peptide was added to the medium on day 9. Neurons were left untreated or subjected to rotenone treatment (5–100 nM for 2 h, diluted in PBS), rinsed, fixed and directly stained for neuronal marker (βIII-tubulin) and mitochondria (Tom20, Santa Cruz Biotechnology). Confocal pictures were taken and blinded to the investigator before image analysis. The sizes of mitochondria in all neuronal extensions of randomly selected neurons were determined using ImageJ software and mitochondria were classified in size categories (ranging from <2 μm to >8 μm). Each category was expressed as percentages relative to the size of the total mitochondrial network for a given neuron. How to cite this article: Szelechowski, M. et al. A viral peptide that targets mitochondria protects against neuronal degeneration in models of Parkinson’s disease. Nat. Commun. 5:5181 doi: 10.1038/ncomms6181 (2014).